Nanobatteries in redox-based resistive switches require extension of memristor theory Redox-based nanoionic resistive memory cells are one of the most promising emerging nanodevices for future information technology with applications for memory, logic and neuromorphic computing. Recently, the serendipitous discovery of the link between redox-based nanoionic-resistive memory cells and memristors and memristive devices has further intensified the research in this field. Here we show on both a theoretical and an experimental level that nanoionic-type memristive elements are inherently controlled by non-equilibrium states resulting in a nanobattery. As a result, the memristor theory must be extended to fit the observed non-zero-crossing I – V characteristics. The initial electromotive force of the nanobattery depends on the chemistry and the transport properties of the materials system but can also be introduced during redox-based nanoionic-resistive memory cell operations. The emf has a strong impact on the dynamic behaviour of nanoscale memories, and thus, its control is one of the key factors for future device development and accurate modelling. Resistive switching memories are nanoionic-based electrochemical systems with a simple metal–ion conductor (insulator)–metal structure. These devices exhibit low power consumption, response times in the nanosecond range and scalability down to the atomic level [1] , [2] , [3] . They demonstrate excellent prospects for the application in modern information technology, in particular for novel logical devices [4] and artificial neuromorphic systems [5] . The link [6] between redox-based nanoionic-resistive memories [7] , memristors [8] and memristive devices [9] has further intensified the research in this important area and inspired the introduction of new concepts [10] , [11] , [12] , [13] and material systems [2] , [3] . Efforts are now focused on a microscopic understanding of the physicochemical processes responsible for resistive switching [14] and on meeting the challenges of circuit design [15] . The system properties and the material performance of redox-based nanoionic resistive memory cell (ReRAM) devices are modulated by quantum effects, excess surface free energy of atomic clusters and nonlinear mesoscopic transport phenomena, owing to the nanodimensions of the devices in both lateral and vertical direction, that are often comparable to space charge layer lengths. The borders of well-known definitions, such as those for ion conductors and insulators, become blurred at the nanoscale, and various classes of materials starting from RbAg 4 I 5 , AgI (as bulk ion conductors) and continuing to SiO 2 and Ta 2 O 5 (as bulk insulators) are all used and termed ionic or mixed ionic–electronic electrolytes at room temperature [16] , [17] , [18] , [19] , [20] . The cation-migration-based electrochemical metallization memory (ECM) cells are a class of ReRAMs that use Ag or Cu as an active electrode and, for example, Pt, Ir or W as an inert counter electrode. A variety of oxide, chalcogenide and halide thin films have been suggested for the solid electrolyte [2] . Applying a positive voltage between the active and the counter electrode leads to an oxidation (dissolution) of the active electrode’s material and to a deposition of metal (Ag or Cu) at the counter electrode. Owing to the high electric field in the order of 10 8 V m −1 , the metallic deposit propagates in a filamentary form and short circuits the cell, thus defining a low-resistive ON state. The filament can be dissolved by applying a voltage of opposite polarity to return the cell to a high-resistive OFF state. The anion-migration-based valence change cells (VCM) typically use a high work function electrode (for example, Pt and TiN), an oxygen-affine, lower work function electrode and a metal oxide as the electrolyte. These cells rely on the formation of oxygen-deficient, mixed ionic–electronic conducting filaments and the nanoionic modification of the potential barrier between the tip of the filament and the electrode to define the ON and OFF states. The ON and OFF states are then used to read the Boolean 1 and 0, respectively. The functionality of ReRAM cells and the kinetics of the filament formation/dissolution are the subject of intensive studies from both, academia and industry, leading to a development of empirical or semi-empirical models for the operating principles [21] , expanding to include concepts of multibit memories [22] and memristive systems [6] , [10] , [15] . From the circuit theory’s point of view, ReRAM cells are regarded as memristive elements or real memristors [23] . They are defined by two simple equations, the state-dependent Ohm’s law, and the state equation The distinctive feature of memristive elements is a pinched characteristics at the origin of the I–V plane (that is, the I–V zero-crossing property) [8] , [9] , which is a direct result of these equations, and therefore represents the essential fingerprint [23] . A short excursus on the use of the term ‘memristor’ is given in Supplementary Note 1 . Here, we report on non-equilibrium ON and OFF states in ReRAM cells determined by chemical potential gradients generating an electromotive force of up to a few hundred millivolts, violating the zero-crossing property. The emf may affect the retention time, and both influences and is influenced by the processes during formation and rupture of the metallic filament. We introduce additional equations to account for the emf, that is, for the non-zero-crossing hysteresis loop, thus qualitatively and quantitatively extending the memristor theory. The conclusions we draw with respect to a series of ECM systems apply to VCM-type ReRAM cells as well as other electrochemical and (neuro-)biological systems. Origins of electromotive force in ReRAM cells To clearly identify the individual influences of different chemical potential gradients, we studied ECM cells build from a series of materials, selected so as to ensure a transition of particular chemical and transport properties, that is, SiO 2 –GeS x , GeSe x –AgI (with x =2.2 and 2.3, respectively). In the as-deposited state, all materials are electronic insulators where the first and the last compounds of this series represent the two extremes. That is to say, SiO 2 has a very small (but at the nanoscale not completely negligible) electronic conductivity and AgI is a stoichiometric ionic compound with considerable Ag + ion conductivity. Neither is able to dissolve Ag chemically. In contrast, GeS x and GeSe x are able to dissolve Ag (or Cu) to different extents moving from insulators to mixed ionic–electronic electrolytes, thus displaying a transport property transition between SiO 2 and AgI. We found three factors that contribute to the formation of the cell voltage V emf , as illustrated in Fig. 1 : (1) the classical Nernst potential V N ( Fig. 1a ), (2) the diffusion potential V d ( Fig. 1b ) and (3) the Gibbs–Thomson potential due to the different surface free energies of macro- and nanoparticles V GT ( Fig. 1c ), for the case that a metallic nanofilament is formed without short-circuiting the electrodes. Note that in the case that a metallic nanofilament is formed, the measureable emf is zero owing to the short circuit ( Fig. 1d ). 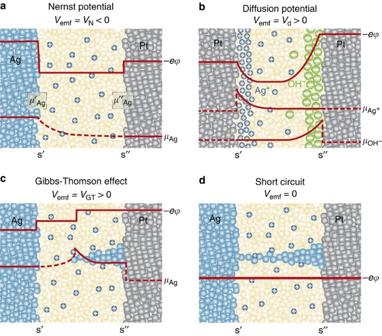Figure 1: Origins of emf in nanoscale cells. These sketches show situations for SiO2-based cells in which one of the three basis origins of emf dominates. (a) A Nernst potentialVNof a Ag/SiO2/Pt cell arising from the difference of the chemical potential of Ag metal at the interfaces Ag/electrolyte and Pt/electrolyte ΔμAg=μ′Ag−μ″Ag. The Nernst potentialVNaccording to equation (11) has a negative value and it is given by the difference of the electrical potentials at both electrodesgenerated to keep the condition(is the electrochemical potential given by). Depending on the specific chemical redox system and the chemical potential gradients, the sign of theVemfcan also be positive. (b) A diffusion potentialVdis generated in a Pt/SiO2/Pt cell by gradients of the chemical potentials of the Ag+and OH−ions, that is,ΔμAg+=μ′Ag+−μ′′Ag+andΔμOH-=μ′ΟΗ-−μ′′ΟH-inhomogeneously distributed in the thin film as given by equation (5). (c) In the case of a nanosize filament, the chemical potential of Ag contains an additional surface energy term generating a chemical potential gradient ΔμAg=μAg-micro−μAg-nanoin accordance with equation (6) (Gibbs–Thomson PotentialVGT). (d) In the case of a fully metallic contact or a highly conducting tunnel junction, the emf isVcell=0. The potential of the right electrode is used as a reference throughout the text. Please note that profiles of the electrostatic potentialφis sketched without zooming into the space charge layers. Figure 1: Origins of emf in nanoscale cells. These sketches show situations for SiO 2 -based cells in which one of the three basis origins of emf dominates. ( a ) A Nernst potential V N of a Ag/SiO 2 /Pt cell arising from the difference of the chemical potential of Ag metal at the interfaces Ag/electrolyte and Pt/electrolyte Δ μ Ag = μ ′ Ag − μ ″ Ag . The Nernst potential V N according to equation (11) has a negative value and it is given by the difference of the electrical potentials at both electrodes generated to keep the condition ( is the electrochemical potential given by ). Depending on the specific chemical redox system and the chemical potential gradients, the sign of the V emf can also be positive. ( b ) A diffusion potential V d is generated in a Pt/SiO 2 /Pt cell by gradients of the chemical potentials of the Ag + and OH − ions, that is, Δ μ Ag + = μ ′ A g + − μ ′ ′ Ag + and Δ μ OH - = μ ′ Ο Η - − μ ′ ′ Ο H - inhomogeneously distributed in the thin film as given by equation (5). ( c ) In the case of a nanosize filament, the chemical potential of Ag contains an additional surface energy term generating a chemical potential gradient Δ μ Ag = μ Ag-micro − μ Ag-nano in accordance with equation (6) (Gibbs–Thomson Potential V GT ). ( d ) In the case of a fully metallic contact or a highly conducting tunnel junction, the emf is V cell =0. The potential of the right electrode is used as a reference throughout the text. Please note that profiles of the electrostatic potential φ is sketched without zooming into the space charge layers. Full size image The Nernst voltage V N is given by the difference between the potential-determining half-cell reactions at each electrode/electrolyte interface: with V s′ and V s″ being the half-cell potentials at the active electrode/electrolyte (s′) and inert electrode/electrolyte (s″) interfaces, z the number of exchanged electrons and V 0 the difference in the standard potentials of these reactions. At the s′ interface, the potential-determining reaction is the same for all ECM cells: At the s″ interface, Red and Ox are general expressions in equation (3) for a species undergoing a redox process. The nature of this species is determined by the specific cell, as will be shown below. The non-equilibrium diffusion potential V d in ECM cells arises owing to excess concentrations of charged species, that is, Ag + ions, electrons and/or OH − ions within the electrolyte film. These ions are introduced into the solid films either electrochemically during forming or SET/RESET cycles or chemically owing to a chemical dissolution of Ag. In both cases, the ratio of concentration changes across the electrolyte layer, with particularly pronounced changes in the vicinity of the electrodes. The electromotive force generated by this inhomogeneous charge distribution and mobilities is given by [24] : where k , T and e are the Boltzmann constant, the temperature and the elementary charge, respectively. and a denote the averaged transference number and the activity of the metal cations, respectively. The averaged transference number and the activity of negatively charged species (anions and electrons) are expressed by and a − . z i is the charge number of each species. The interfaces denoted by s′ and s″ correspond to the active electrode/electrolyte and the inert electrode/electrolyte interfaces, respectively. The potential difference generated in the neuron cells to transport electric signals has the same nature and originates in the diffusion (Donnan) potential [24] . The contribution of the third component V GT to the total cell voltage V emf is expected in the case of a non-contacting filament owing to the different surface free energies of the macrocrystalline active electrode and the nanosize filament in accordance with the Gibbs–Thomson equation: where γ is the surface free energy, r is the radius of the particle, V m is the molar volume and μ Ag is the chemical potential of Ag. V GT can be observed, for instance, for high-resistive ( R >12.9 kΩ) ON states (no metallic short circuit) typically caused by filaments in ECM cells without galvanic contact to the active electrode (see Supplementary Fig. S1 ). It should be noted that the contribution of V GT could not be clearly distinguished from the contribution of V d in the particular systems we have studied. ReRAM cells based on initially insulating thin films In Fig. 2 , we show the time evolution of the open cell voltage V cell and of the short circuit current I for Ag/SiO 2 /Pt cells. 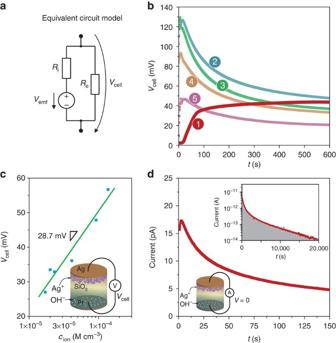Figure 2: Steady-state emf measurements for Ag/SiO2/Pt ECM cells. (a) Simplified equivalent circuit model of a ReRAM device. (b)Vcellfor a Ag/SiO2/Pt cell measured under open circuit conditions. The red line curve (1) depictsVcellin the OFF state after a SET/RESET cycle. For the other curves, the ion concentrationcion(that is, the sum of the Ag+and OH−ion concentrations, averaged over the thickness) was controlled and preset using different sweep rates25. Curve (2) corresponds tocion=1.4 × 10−4M cm−3, (3) tocion=9.2 × 10−5M cm−3, (4) tocion=2 × 10−5M cm−3and curve (5) tocion=1.7 × 10−5M cm−3, respectively. Details of the measurements are depicted inSupplementary Fig. S2. Further voltage sweeps in the negative voltage regime result in further decrease of the ion concentration (Supplementary Fig. S3). (c) The slope of the line provides the pre-exponential term and we were thus able to determine the ionic transference numberby using equations (10) andz=+1 (for Ag+). (d) The time evolution of the discharge current (forV=0 V) of the cell (diameterd=100 μm) after SET and subsequent RESET operation is shown. Inset: the same plot for an extended time and a log current scale. The integration reveals the charge (5 nC) of the nanobattery. Figure 2a displays the simplified equivalent circuit of the nanobattery where the cell voltage is Figure 2: Steady-state emf measurements for Ag/SiO 2 /Pt ECM cells. ( a ) Simplified equivalent circuit model of a ReRAM device. ( b ) V cell for a Ag/SiO 2 /Pt cell measured under open circuit conditions. The red line curve (1) depicts V cell in the OFF state after a SET/RESET cycle. For the other curves, the ion concentration c ion (that is, the sum of the Ag + and OH − ion concentrations, averaged over the thickness) was controlled and preset using different sweep rates [25] . Curve (2) corresponds to c ion =1.4 × 10 −4 M cm −3 , (3) to c ion =9.2 × 10 −5 M cm −3 , (4) to c ion =2 × 10 −5 M cm −3 and curve (5) to c ion =1.7 × 10 −5 M cm −3 , respectively. Details of the measurements are depicted in Supplementary Fig. S2 . Further voltage sweeps in the negative voltage regime result in further decrease of the ion concentration ( Supplementary Fig. S3 ). ( c ) The slope of the line provides the pre-exponential term and we were thus able to determine the ionic transference number by using equations (10) and z =+1 (for Ag + ). ( d ) The time evolution of the discharge current (for V =0 V) of the cell (diameter d =100 μm) after SET and subsequent RESET operation is shown. Inset: the same plot for an extended time and a log current scale. The integration reveals the charge (5 nC) of the nanobattery. Full size image Here, t ion represents the total ionic transfer number, R i is the total resistance of the ionic current path and R e the total electronic resistance of the cell. Figure 2b shows V cell after establishing a defined concentration c ion of Ag + and OH − ions for unformed cells. We utilized the fact that the amount of ions generated at the s′ and s″ interfaces during cell operation is adjusted by the pulse length and height or the sweep rate [25] . The decrease of V cell over a few hundred seconds is caused by the equilibration of the Ag + and OH − concentration gradient, which has an initial maximum immediately at the metal/electrolyte interface. Furthermore, Fig. 2b (red line) shows V cell immediately after a RESET operation and switching to the open cell measuring conditions. In this case, the Ag + concentration in the immediate vicinity to the Ag electrode is depleted (in contrast to unformed cells) on the one hand side owing to the reduction process (that is, the RESET process) and on the other hand side owing to slow supply/diffusion of ions from layers apart from the interface (diffusion limited). Thus, in this situation V cell increases with time but relaxes to the same value as the unformed cells after equilibration. The potential-determining reaction at the inert electrode, for example, Pt, depends on the material properties of the solid electrolyte and we distinguish two cases. The system Ag/SiO 2 /Pt represents the first case for which the solid SiO 2 film contains no initial Ag + and, hence, reaction (4) cannot be potential-determining. Instead, as shown in Tsuruoka et al . [26] , moisture is typically incorporated into this electrolyte during fabrication and hence protons provide the required counter reaction at the inert electrode, for example, and the Nernst voltage takes the form: The total emf of the ECM cell is a combination of equations (5) and (9) and is expressed by: with V 0 = V 0 +const. (see Supplementary Note 2 ). In Fig. 2c we evaluate V cell after initial relaxation. The slope of the line provides the pre-exponential term and we were thus able to determine the ionic transference number by using equation (10). The x -axes intercept corresponds to the condition ln( a ion )=0 and provides the value of V 0 =0.17 V. Both values are used as parameters in the device modelling below. Figure 2d illustrates the short-circuit currents of a Ag/SiO 2 /Pt cell after RESET operation. In the inset, an extended discharge time of 20,000 s (~5.5 h) is shown. The measurements were carried out until they approached the resolution limit of our measuring system (~10 fA). The current is proportional to the electrode area (see Supplementary Fig. S4 ). An integration of current over time reveals a total charge of ~5 nC released during the discharge of the battery, which corresponds to a conversion of ~2 monolayers Ag. In comparison, the dielectric discharge of the cell capacitor is ~0.4 pC, clearly demonstrating that the discharge phenomenon is of an electrochemical nature. Please note that retention time of the cell (here: in the OFF state) is not immediately related to the relaxation time of the emf voltage. While the first has to be >10 years for universal non-volatile memories, the latter may be in the order of minutes to days as shown. In other words, the discharge of the ReRAM nanobattery does not lead to a loss of the OFF state (in a similar manner as the discharge of any other rechargeable battery does to end up in a filamentary short between the electrodes). Instead, typically only a shift of the particular R OFF value is observed upon the relaxation of the emf. Such a shift has been reported, for example, by Miao et al . [27] and Choi et al . [28] for both ECM and VCM systems, respectively. More detailed discussion is provided in Supplementary Note 3 . ReRAM cells based on mixed conducting thin films In the second case condition for establishing a Nernst voltage according to equation (3), the electrolyte contains mobile Me z + ions dissolved by electrochemical and/or chemical processes with almost homogeneous distribution, that is, ( a MML:Me z + ) s′ ~( a MML:Me z + ) s″ . Then the potential-determining half-cell reaction at the s″ interface will be the same as at s′, that is, reaction (4), and, because no chemical potential gradient of the charged species is assumed, equation (3) can be simplified to: where ( a Me ) s′ denotes the activity of the active metal Me at interface s′, that is, ( a Me ) s′ =1, if a pure metal is used, and ( a Me ) s″ is the activity of Me at the inert counter electrode s″, that is, ( a Me ) s″ is typically very low. is the ion transference number averaged throughout the electrolyte thickness. As ( a Me ) s′ is fixed, the Nernst voltage is a function of ( a Me ) s″ alone. We succeeded in demonstrating a Nernst emf in accordance with equation (11) ( Fig. 1a ) for the systems Ag/Ag–GeS 2.2 /Pt and Ag/Ag–GeSe 2.3 /Pt, which contain a significant amount of chemically dissolved Ag + ions (a solubility of up to 35 at% Ag has been reported [29] ). We applied a positive external voltage of 1 V to the inert electrode, thus removing the residual Ag atoms from the s″ interface and lowering their activity. In the coupled cathodic reaction at the Ag interface s′, Ag dendrites are deposited as shown in the optical image in Fig. 3 . Thus, apart from the different concentration of Ag + ions at both interfaces, we generated a difference in the activities of Ag. The emf of the system was then monitored over time and correlated to the evolution of the dendrite morphology further recorded by optical images. The time evolution shown in Fig. 3 arises from the interplay of a Nernst potential and a diffusion potential. In the voltage-modified state ( t 1 in Fig. 3 ), the contribution of the (positive) diffusion potential fades, leading to a dominating (negative) Nernst potential, which results to an emf value of ~−450 mV owing to the contribution of equation (11). The emf value corresponds to a difference in the Ag activities at both electrodes, ( a Ag ) s″ ≈2.5 × 10 −8 ( a Ag ) s′ . As monolayer(s) of Ag begin to form at the Pt electrode (in parallel to the dissolution of the dendrites at the Ag electrode), the emf increases again simultaneously and relatively fast because of ( a Ag ) s′ ≈ ( a Ag ) s″ . But owing to slower diffusion of the Ag + ions a (Ag + ) s′ > a (Ag + ) s″ the positive diffusion potential governs V cell . Thus, the control over V cell changes from a situation mainly determined by equation (11) to a situation dominated by equation (5). 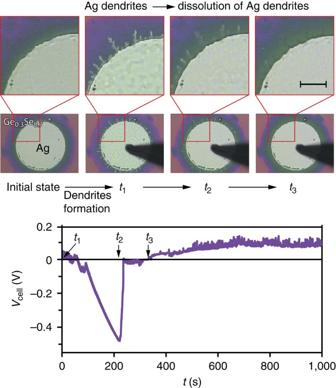Figure 3: Time-dependent emf measurements for Ag/Ge0.3Se0.7/Pt ECM cells. After a SET/RESET cycle (initial state), a negative voltage is applied to the Ag electrode resulting in a dendrite formation. Att1=0 s the voltage measurement is started. Fading of the diffusion potential contribution fromt1tot2leads to a highly negativeVcellowing to a significant Nernst potential between the electrodes. In parallel to the dissolution of the dendrites (t2), the emf increases to positive values again with a diffusion potential as the remaining component of the emf owing to the different activity of Ag+ions at the both s′, s″ surfaces (t>t3). The scale bar in the inset corresponds to 20 μm. Figure 3: Time-dependent emf measurements for Ag/Ge 0.3 Se 0.7 /Pt ECM cells. After a SET/RESET cycle (initial state), a negative voltage is applied to the Ag electrode resulting in a dendrite formation. At t 1 =0 s the voltage measurement is started. Fading of the diffusion potential contribution from t 1 to t 2 leads to a highly negative V cell owing to a significant Nernst potential between the electrodes. In parallel to the dissolution of the dendrites ( t 2 ), the emf increases to positive values again with a diffusion potential as the remaining component of the emf owing to the different activity of Ag + ions at the both s′, s″ surfaces ( t>t 3 ). The scale bar in the inset corresponds to 20 μm. Full size image Emfs for different types of VCM and ECM memory cells In the course of our emf studies, we investigated a series of different ECM cells as well as selected VCM cells. We were able to prove that in all types of ReRAM cells tested significant (electro)chemical potential gradients are generated by the operation of the cells. Inevitably, these gradients give rise to an emf, and, hence, the cells show the characteristics of nanosize batteries with cell voltages in the range displayed in Fig. 4a (for details see Supplementary Table S1 ). After forming, the cell voltages of VCM cells are much lower than for ECM cells owing to the significantly higher electronic conductance in the OFF state originating from the stub of the highly conductive filament. 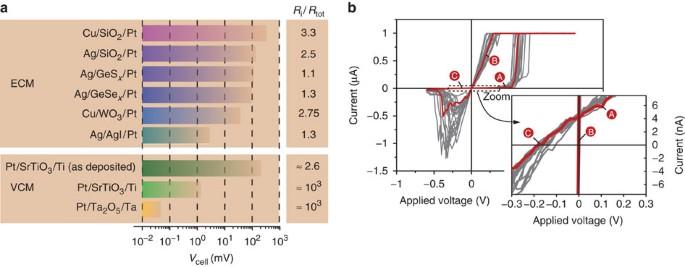Figure 4: Emf for different types of ReRAM cells. All tested cells showed an emf varying from some hundreds of microvolts to some hundreds of millivolts (a). The specific steady-state emf depends on the type of cell and the device operation (for example, sweep rate or voltage amplitude before the (open cell) emf measurement). For the sake of completeness, the internal resistanceRinormalized by the total resistanceRtotis given (for details: seeSupplementary Table S1). The influence of the emf on the current–voltage sweeps, resulting in non-zero-crossing characteristics (b), is given for the Cu/SiO2/Pt system (red curve) as an example (electrode areaAcell=2 × 10−4cm2, sweep rateν=400 mV s−1). TheI–Vcharacteristics in grey are provided for statistical verification. For the sake of clarity, the currents of the OFF state (A) and (C) and the ON state (B) are labelled, respectively. The formed valence change memory (VCM)-type cells (Ti/SrTiO3/Pt and Ta/Ta2O5/Pt) show lower emf for the OFF state owing to the higher electronic partial conductivity, that is, higher currents, but lower ion transference number. Emfs for VCM cells are depicted inSupplementary Figs S7,S8, respectively. TheI–Vcharacteristics for Ag/SiO2/Pt and Ti/SrTiO3/Pt cells are shown inSupplementary Figs S9,S10. Figure 4: Emf for different types of ReRAM cells. All tested cells showed an emf varying from some hundreds of microvolts to some hundreds of millivolts ( a ). The specific steady-state emf depends on the type of cell and the device operation (for example, sweep rate or voltage amplitude before the (open cell) emf measurement). For the sake of completeness, the internal resistance R i normalized by the total resistance R tot is given (for details: see Supplementary Table S1 ). The influence of the emf on the current–voltage sweeps, resulting in non-zero-crossing characteristics ( b ), is given for the Cu/SiO 2 /Pt system (red curve) as an example (electrode area A cell =2 × 10 −4 cm 2 , sweep rate ν =400 mV s −1 ). The I–V characteristics in grey are provided for statistical verification. For the sake of clarity, the currents of the OFF state (A) and (C) and the ON state (B) are labelled, respectively. The formed valence change memory (VCM)-type cells (Ti/SrTiO 3 /Pt and Ta/Ta 2 O 5 /Pt) show lower emf for the OFF state owing to the higher electronic partial conductivity, that is, higher currents, but lower ion transference number. Emfs for VCM cells are depicted in Supplementary Figs S7,S8 , respectively. The I – V characteristics for Ag/SiO 2 /Pt and Ti/SrTiO 3 /Pt cells are shown in Supplementary Figs S9,S10 . Full size image The non-equilibrium states reflected by the emf voltage may affect both the retention and the device operation. Although OFF and intermediate states always experience emf voltages, for ON states with metallic contact the cell voltage is generally close to zero owing to the electronic conductance of the filament. Apart from that, chemical potential gradients, size effects and electrolyte non-stoichiometry can result in a chemical dissolution of the filament [30] . Thus, the retention of the ON state is strongly dependent on the filament characteristics and only indirectly dependent on the emf voltage. Being an intensive state property, V emf is independent on the cell size. However, the ionic and electronic resistances, R i and R e , and hence V cell may scale in a non-trivial manner depending on the ReRAM type, for example, the properties of the filament stub and the gap between the filament tip and the electrode in the case of VCM cells. This is further illustrated in Supplementary Figs S5,S6 . Our results strongly suggest that in all bipolar ReRAM devices a nanobattery with dedicated emf voltages is present. This fact has far-reaching consequences on the application of the theory of memristive elements and on the device modelling in general. The emf is a state property corresponding to a non-zero-crossing I–V characteristic (compare Fig. 4b ), and we correspondingly expanded the memristive equations to obtain an active device that can be considered an extended memristive element. In fact, any electrochemical system is active by nature, thus two-terminal nanoionic-resistive switches cannot be pure passive memristors. The same is true for neurobiological systems, which are also active, offering passive memristive elements only as internal elements [31] . However, in contrast to the emf of ReRAM cells, the biological resting membrane potential is modulated only by V d (eq. (5)) and not by V N (eq. (3)). By abandoning the zero-crossing property, a large number of dynamical devices can be added to the framework of memristive, memcapacitive and meminductive devices. For example, ferroelectric capacitors as well as ferromagnetic inductors can thus be regarded as extended memcapacitive and meminductive elements, respectively ( Fig. 5a ). By means of this expanded framework, a ReRAM cell is still a memristive device, as shown in Fig. 5a . 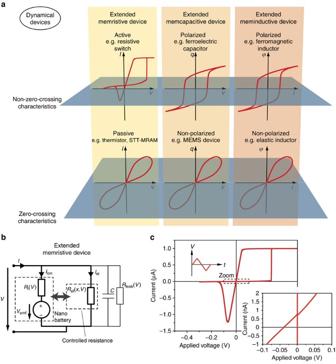Figure 5: Classification of mem devices. (a) Memristive, memcapacitive and meminductive devices are assumed to offer pinched characteristics at the origin in general39. In the case of memcapacitive and meminductive devices, a spontaneous polarization of a ferroelectric and ferromagnetic material, respectively, leads for example, to non-zero-crossing characteristics11. Similarly, a non-zero-crossingI–Vcharacteristic of a memristive device indicates the presence of an inherent nanobattery, that is, this device is active. Therefore, we introduce the generic terms extended memristive device, extended memcapacitive device and extended meminductive device to account for both zero-crossing and non-zero-crossingI–Vcharacteristics. Note that the origin of non-zero-crossing behaviour in memcapacitive and meminductive devices is of completely different nature than in memristive devices, thus require specific modifications of the concept. Interestingly, spin-transfer torque (STT) MRAM cells offer zero-crossing in contrast to ReRAM cells, thus can be considered as conventional memristive device. (b) Equivalent circuit of the extended memristive element. The ionic current is defined by the nanobattery, which controls the state-dependent resistor representing the electronic current path. The capacitance of the device is neglected as its influence is not significant. The partial electronic conductivity in the electrolyte induces a state-independent resistanceRleakdue to a leakage current in parallel. (c) SimulatedI–Vcharacteristic of the extended memristor. The zoom shows the non-zero-crossing behaviour. Further considerations on the simulation are described inSupplementary Note 4. Figure 5: Classification of mem devices. ( a ) Memristive, memcapacitive and meminductive devices are assumed to offer pinched characteristics at the origin in general [39] . In the case of memcapacitive and meminductive devices, a spontaneous polarization of a ferroelectric and ferromagnetic material, respectively, leads for example, to non-zero-crossing characteristics [11] . Similarly, a non-zero-crossing I – V characteristic of a memristive device indicates the presence of an inherent nanobattery, that is, this device is active. Therefore, we introduce the generic terms extended memristive device, extended memcapacitive device and extended meminductive device to account for both zero-crossing and non-zero-crossing I – V characteristics. Note that the origin of non-zero-crossing behaviour in memcapacitive and meminductive devices is of completely different nature than in memristive devices, thus require specific modifications of the concept. Interestingly, spin-transfer torque (STT) MRAM cells offer zero-crossing in contrast to ReRAM cells, thus can be considered as conventional memristive device. ( b ) Equivalent circuit of the extended memristive element. The ionic current is defined by the nanobattery, which controls the state-dependent resistor representing the electronic current path. The capacitance of the device is neglected as its influence is not significant. The partial electronic conductivity in the electrolyte induces a state-independent resistance R leak due to a leakage current in parallel. ( c ) Simulated I – V characteristic of the extended memristor. The zoom shows the non-zero-crossing behaviour. Further considerations on the simulation are described in Supplementary Note 4 . Full size image The starting point for a practical memristive model of a ReRAM cell is the memristive model from Strukov et al . [6] , to which we add the nanobattery in parallel. The resulting model, which we term an extended memristive model, consists of a voltage source V emf and a nonlinear internal resistance R i —which together form the nanobattery—and a parallel resistor R el whose state variable x is controlled by the nanobattery ( Fig. 5b and Supplementary Fig. S11 ). The state-dependent resistance of the electronic current path ( R el ) is a nonlinear function of the applied voltage, for example a tunnelling equation [32] . The electronic leakage current is accounted by a further parallel resistance R leak , which is state-independent and already present in the pristine device. Both contributions, R el and R leak , in parallel represent R e in Fig. 2a . The resistance of the ionic current path ( R i ) is defined by another nonlinear equation, determined by the Butler–Volmer equation and/or the high-field drift equation. The state-dependent Ohm’s law for the extended memristive device reads: and the state equation (compare Fig. 5b ) reads: where d is the thickness of the active layer and K 1 is a constant while I ion offers a highly nonlinear voltage dependence, responsible for the pronounced nonlinearity of the switching kinetics. To fit the observed changes in the emf measurements ( Fig. 2 ), a second-state variable, the ion concentration c ion , is required. In this case, the emf equation (10) with the experimentally determined V 0 =0.17 V for Ag/SiO 2 /Pt ( Fig. 2c ) reads: Modelling details are described in the Supplementary Note 4 and corresponding simulation results are depicted in Fig. 5c . The inset clearly shows the non-zero-crossing I–V behaviour. Thus, ReRAM cells are non-zero-crossing devices, and therefore, the original memristor theory must be significantly extended in order to accommodate redox-based resistive switching systems. Besides modelling accuracy, the emf also has direct impact on future memory device development and corresponding circuitry. First, the stability of intermediate resistive states (for example, required in multilevel memory and neuromorphic applications) must be carefully considered in terms of the emf. Moreover, the effect of the emf within ultra-dense passive crossbar arrays may become relevant owing to possible device-to-device interactions. Second, the READ voltage of future generation memory elements will be in the range of 100 to 200 mV (ref. 33 ). This voltage is in the same order of magnitude as the emf voltage of some of the ReRAM types studied here. Third, the READ current for a ReRAM cell in a memory matrix will be in order of 100 nA and the length of the READ pulse <100 ns. Hence, during the READ operation, a total charge of Q =100 nA × 100 ns=10 fC will be transferred to or from a memory cell. As shown in our paper, the total nanobattery capacity for scaled ReRAM cells may easily be in the same order of magnitude or higher. These points demonstrate impressively the relevance of nanobattery effect for the performance and reliability of future ReRAM devices, and the necessity of including it in the device modelling. Apart from that, the emf allows for novel read-out approaches in ReRAM cells, for example, we suggested using the emf for non-destructive read-out of complementary resistive switches [34] . The theoretical implication has been raised in refs 35 , 36 . In conclusion, we found clear indications that non-equilibrium states occur in nanoionic ReRAM cells, which are generated by chemical processes such as the dissolution of the active electrode material into the electrolyte, by electrochemical processes and by charge redistribution during the operation of the cells. The resulting electromotive force suggests the presence of a nanobattery inside the memristive device as an inherent property of the system. The nature of ReRAM systems implies a mandatory extension of the memristor theory, in order to include the non-zero-crossing characteristics. Sample preparation All samples were prepared using platinised silicon wafers as substrates. The solid electrolytes/insulators were deposited on the substrate using e-beam or thermal evaporation or radio frequency (RF) sputtering. SiO 2 . Thirty nanometre to 50-nm SiO 2 films were deposited by electron beam evaporation at 10 −4 Pa at a deposition rate of 0.01 nm s −1 . Later, pattern transfer of top microelectrodes with a diameter of 100 to 250 μm was done using conventional UV lithography. Ag (Cu) with a thickness of 30 nm was deposited by e-beam evaporation (evaporation speed 0.025 nm s −1 ) followed by a 100-nm-thick DC-sputtered Pt layer to prevent chemical oxidation of the silver (copper) electrode in air. WO 3− x . Thirty-nanometre WO 3− x films were sputtered in Ar plasma at a pressure of 10 Pa with an RF power of 121 W, using a WO 3 target. Subsequently, 70-nm-thick Cu electrodes 50 μm in diameter (UV lithography) were thermally evaporated. GeS 2.2 . Fifty-nanometre GeS 2.2 films were deposited by RF sputtering at a gas flow of 50 s.c.c.m., 20 Pa Ar pressure and RF power of 20 W. The S/Ge ratio was determined by EDX (Oxford Instruments ISI 300, at 20 kV acceleration voltage). Ag electrodes, microstructured by UV lithography, with diameters between 10 and 100 μm and a thickness of 100 nm were RF sputtered at a gas flow of 50 s.c.c.m., RF power of 50 W and 20 Pa pressure. The relatively high pressure in the deposition chamber allows the deposition of homogeneous thin films [37] . GeSe 2.3 . Fifty to 70-nm GeSe 2.3 films were sputtered at a gas flow of 40 s.c.c.m., process pressure of 7 × 10 −2 Pa and RF power of 13 W. The deposition rate was 0.075 nm s −1 . The preparation of the electrodes is identical to that described for GeS 2.2 . AgI. Thirty to 50-nm AgI films were prepared by thermal evaporation. To avoid any impact of UV light and chemicals, the pattern transfer for the top electrode was done directly after subtractive pattern transfer of the Pt bottom electrode using reactive ion etching. A detailed description of the fabrication of Ag/AgI/Pt cells can be found in Tappertzhofen et al . [18] SrTiO 3 . Seventy nanaometre of Ti was sputtered in argon plasma at an RF power of 20 W, a pressure of 0.8 Pa and a substrate temperature of 200 °C, followed by the application of 8 nm of SrTiO 3 , using the same process parameters and a sintered ceramic target. The Pt top electrodes with a thickness of 30 nm were sputtered at a pressure of 0.8 Pa and RF power of 12 W for lower kinetic impact. All layers were deposited without breaking the vacuum to prevent contamination. Ta 2 O 5 . Fifty nanaometre of Ta was sputtered in argon plasma at an RF power of 14 W, a pressure of 0.8 Pa and a substrate temperature of 200 °C. Subsequently, the Ta layer was oxidized using an argon–oxygen atmosphere with a ratio of 3:1 and an oxygen partial pressure of 100 Pa, forming a Ta 2 O 5 surface layer with a thickness of 15–20 nm. The Pt top electrodes with a thickness of 30 nm were sputtered at a pressure of 0.8 Pa and RF power of 12 W for lower kinetic impact. All layers were deposited without breaking the vacuum to prevent contamination. Electrical characterization The emf measurements were performed in a four-needle electrode microprobe station equipped with micromanipulators to contact the sample electrodes and an optical microscope to visually monitor the surface. For potentiodynamic current–voltage measurements, we applied triangular voltage sweeps between −1.5 and 1.5 V at various sweep rates (30 mV s −1 to 2 V s −1 ) using a Keithley 6430 sub-femtoampere SourceMeter. Details of the measuring method can be found in refs 25 , 38 . Electromotive forces were measured using the 6430 SourceMeter with high input impedance (>10 14 Ω), a Keithley 617 electrometer (>200 TΩ) and a Keithley 2636A SourceMeter (>10 14 Ω) for comparison. Throughout the paper, the right electrode in cells denoted M′/I/M′′ was used as reference electrode for all measurements. We used triaxial cables and electrostatic shielding to avoid RFI effects. The offset voltage measured across a 10 MΩ resistor has been proven to be within the device specification (below 1 μV accuracy). Details on the measurement resolution and accuracy are shown in Supplementary Fig. S12 and Supplementary Table S2 , respectively. How to cite this article: Valov, I. et al . Nanobatteries in redox-based resistive switches require extension of memristor theory. Nat. Commun. 4:1771 doi: 10.1038/ncomms2784 (2013).